Effective impedance boundary optimization and its contribution to dipole radiation and radiation pattern control Radiation pattern control has generated much interest recently due to its potential applications. Here we report the observation of high-efficiency dipole-like radiation of sound with broad bandwidth through a decorated plate with periodical two-dimensional Helmholtz resonators on both sides and a single slit at the centre. The decorated plate was optimally designed to adjust the effective impedance of the boundary, and the underlying mechanism of radiation pattern control is attributed to wave vector tailoring. The high radiation efficiency is due to the Fabry–Perot resonances associated with waveguide modes in the centre slit. The method to obtain a collimated beam without any sidelobes is also provided. Our findings should have an impact on acoustic applications. Owing to diffraction effects, waves diverge when propagating in a homogeneous medium. However, in practical applications, omnidirectional radiation is not always welcomed. Controlling and modulating different radiation patterns in different practical applications will not only save the transmission energy but also keep the transmitted signal confidential. Horn and phased arrays are two different approaches to obtain different kinds of radiation patterns. The underlying mechanism is to utilize the interference—for example, the waves emitted from all points on the Airy beam profile—in order to maintain a propagation-invariant Airy structure [1] , [2] , [3] . Perhaps the best known example of such an approach is the one used to obtain a Bessel beam pattern [4] . Recent progress in the research area of photonic and phononic crystals and metamaterials provides a new approach to realize radiation pattern control and modulation. Early studies focused on spatial dispersion affected by spatial periodicity to modulate radiation patterns—that is, utilizing crystal anisotropy to counteract the spreading of the wave [5] , [6] , [7] —and band-edge states are the most important factors for realizing it [8] , [9] , [10] . Recently, based on the form-invariant form of Maxwell’s equations under certain coordinate transformations, transformation optics for controlling the electromagnetic fields has proved to be an effective approach for manipulating ray traces [11] , [12] . The successful application of transformation optics to wave modulation in cylindrical coordinates modulates the omnidirectional line radiation source to specified patterns and directions [13] . In addition to radiation pattern control, the modulation of the wave can also produce phenomena such as lensing and hyperlensing [14] , [15] , [16] , [17] . However, these approaches modulate radiation patterns by adjusting the material properties throughout the propagation region. However, for widespread situations, it is impossible to do so. In addition to adjusting the material properties, adjusting the surface impedance may be another effective way to modulate radiation patterns. In electromagnetism, a smooth conducting sheet has low surface impedance. A periodically grooved subwavelength structure in the surface of metal can convert low surface impedance to high surface impedance [18] . However, in acoustics, we would like to convert high acoustic surface impedance to low acoustic surface impedance. Another property of metals is that they support surface waves [19] , but acoustic surface waves do not exist in fluid domain. In this study, in the acoustic scope, we propose a method that utilizes boundaries instead of an entire propagation region to control the radiation pattern, which will greatly reduce the complexity in pattern control and expand the application of wave modulation. Compared with utilizing the interference to control the radiation pattern and realizing waves such as cosine-Bessel beams, utilizing boundaries to control the radiation pattern will greatly reduce the scale of the source. The realization of Bessel beam is through the superposition of an infinite number of plane waves that need a source with large scale [4] ; however, in our proposal, we can control the radiation pattern by utilizing appropriate boundaries with a point source. A system consisting of a single slit surrounded by finite, periodically drilled cavities is designed and fabricated. In this structured system, both the experiment and the numerical calculation demonstrate that the dipole-like radiation pattern can occur over a relatively wide frequency range. It may seem that our system is similar to that of a single slit surrounded by finite, periodically perforated grooves; however, the experimental phenomenon and the mechanism of our system are quite different. The directional beam experimental report by Zhou et al. [20] showed very strong fingerprints of the running surface wave scattered by the grooves [20] , [21] , [22] , and the directional beam occurred in a very narrow bandwidth. We verify that the dipole-like pattern radiation phenomenon in our samples arises from the effective boundary impedance adjustment. The periodically drilled cavity is designed to adjust the effective impedance of the boundary, creating a dipole-like radiation pattern with no sidelobes. Experimental design to obtain dipole-like radiation pattern As shown in Fig. 1a , the decorated sample is a steel plate with periodical two-dimensional (2D) Helmholtz resonators (HRs) on both sides and a single slit at the centre. The thickness of the plate ( t ) and the period of HRs ( d ) are 3.6 mm and 8 mm, respectively. The width of the central slit ( r ) is 2 mm. The total width and height of the decorated sample are 25.8 cm (thereby covering 32 periodical units, with each side containing 16 units) and 25 cm, respectively. The length ( l ) and width ( w ) of the neck of the HRs are 0.5 mm and 1 mm, respectively. The length and the width of the cavity of the HRs ( h ) are both 5 mm. The experiment was carried out in an anechoic chamber in order to eliminate the influence of the reflected waves. 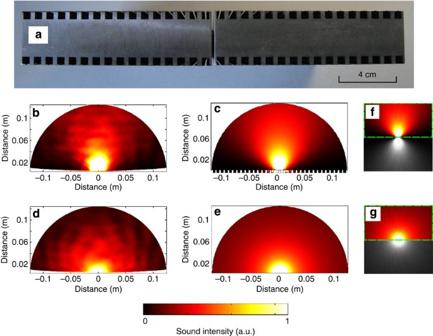Figure 1: Experimental observation of dipole-like radiation pattern. (a) Top views of the sample fabricated by patterning periodical HR on both sides and a single slit at the centre. Scale bar, 4 cm. (b) Experimental and (c) simulated results of intensity patterns of a plane wave passing decorated sample. (d) Experimental and (e) simulated results of intensity patterns of a plane wave passing undecorated sample. (f,g) Simulated intensity patterns for dipole and monopole. The upper half-plane is tagged by the dashed green box for comparison. Figure 1: Experimental observation of dipole-like radiation pattern. ( a ) Top views of the sample fabricated by patterning periodical HR on both sides and a single slit at the centre. Scale bar, 4 cm. ( b ) Experimental and ( c ) simulated results of intensity patterns of a plane wave passing decorated sample. ( d ) Experimental and ( e ) simulated results of intensity patterns of a plane wave passing undecorated sample. ( f , g ) Simulated intensity patterns for dipole and monopole. The upper half-plane is tagged by the dashed green box for comparison. Full size image The full range of the intensity pattern was mapped within an acoustic plane wave normally incident on the decorated sample. A dipole-like radiation pattern without sidelobes is shown in Fig. 1b . The intensity distribution is quite different from that of conventional wave theory. In Fig. 1c , we present the numerical intensity distribution through the finite element method by considering the boundary to be rigid at the surface of the sample due to the large impedance contrast between the air and steel. The numerical results, with no adjustable parameters, are in good accord with the experimental results. Note that the dipole-like radiation phenomenon occurs when the wavelength ( λ =40 mm) is much larger than the period of the HRs ( d =8 mm), which can be utilized to realize device miniaturization. As no sidelobes occur in the pattern, the pattern is not due to the excitation of the acoustic surface wave emerging only in the vicinity of the resonant transmission peak [20] . Actually, the dipole-like radiation pattern can occur in a very wide bandwidth, which is illustrated below. For a better comparison, the experimental and numerical results of the diffraction intensity pattern for the undecorated sample—that is, the sample without HRs—are shown in Fig. 1d,e , respectively. The distribution shows omnidirectional propagation after passing the slit when the scale of the slit is much smaller than the wavelength. This good agreement between the experiment and the simulation illustrates that HRs are the main factor influencing the emergence of the radiation pattern of the acoustic wave. The intensity field of the dipole is shown in Fig. 1f and the half-plane is tagged for comparison. From Fig. 1b,c,f , it is found that the corresponding figures are very nearly identical, showing that the pattern caused by the decorated sample is dipole-shaped. For the undecorated sample, the intensity patterns are very similar to those of the half-plane of a monopole radiation field. The intensity field of the monopole is shown in Fig. 1g for comparison. High-efficiency dipole radiation Intuitively, the radiation efficiency of the dipole radiator is very low—that is, the efficiency of the monopole is proportional to ( k 0 a ) [2] —but for a dipole the efficiency is proportional to ( k 0 a ) [4] , where k 0 and a are the wave number in the host media and the scale of the radiator, respectively. Contrary to expectations, we obtained very high radiation efficiency through the decorated sample (that is, dipole radiation field). In the 3- to 11-kHz interval, two transmission peaks are located at λ =10.2 d ( f =4,224 Hz) and λ =4.9 d ( f =8,832 Hz) for the decorated sample and λ =10.3 d ( f =4,160 Hz) and λ =5.1 d ( f =8,384 Hz) for the undecorated sample. The high radiation efficiency arises from Fabry–Perot resonances associated with waveguide modes in the centre slit [23] . 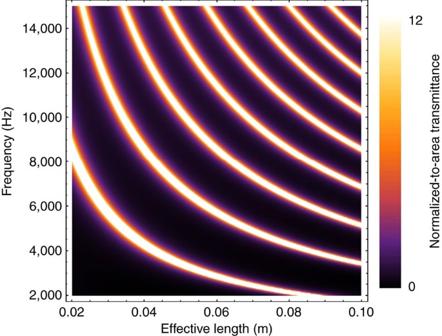Figure 2: Transmittance behaviour. Normalized-to-area transmittance versus the effective length of the centre slit and frequency. At the resonance condition for standing-wave excitation (, in whichmis an integer), transmission enhancement occurs. Figure 2 presents the normalized-to-area transmittance versus the effective length of the centre slit and frequency according to Fabry–Perot resonance theory. At the resonance condition for standing-wave excitation ( , in which m is an integer), transmission enhancement occurs. Here, l 0 = t+ Δ l is the effective length of the centre slit and Δ l is the correction length induced by added acoustical mass due to radiation (see Supplementary Note 1 ). Although the resonance peak is relatively narrow, it should be mentioned that the transmission resonance is utilized to enhance the radiation efficiency. Moreover, the dipole-like radiation pattern can occur in a relatively wide frequency band. If the frequency of the incident wave is not located in the vicinity of the transmission resonance peak, the dipole-like pattern will still occur but with low radiation efficiency. Figure 2: Transmittance behaviour. Normalized-to-area transmittance versus the effective length of the centre slit and frequency. At the resonance condition for standing-wave excitation ( , in which m is an integer), transmission enhancement occurs. Full size image Theory of effective impedance boundary It is known that if a point source is put on an infinity boundary with either a rigid or free boundary, the acoustic field can be regarded as that produced by the source and an imaginary source with the same phase or with an opposing phase in the symmetric position. If the point source is near the boundary, the source and the imaginary source can be regarded as either a monopole or a dipole [24] , [25] . It seems that the undecorated sample will induce the monopole-like fields. For the decorated sample, if the radiation pattern can be attributed to the impedance adjustment by the HRs, thus changing the rigid boundary to be free or quasi-free, the dipole or dipole-like radiation field caused by the decorated sample can be understood. Now an interesting question arises: how the HRs can convert the rigid boundary to a free-boundary condition. To find the underlying mechanism caused by the HRs, we would calculate the effective impedance of the boundary. The boundary condition in the frequency domain is described by specific acoustic impedance, which is defined as . Here, p is the acoustic pressure and v n is the normal particle vibration velocity. Two special circumstances are regarded as free and rigid boundary conditions when Z s →0 and Z s →∞, respectively. On a subwavelength scale, the specific acoustic impedance formulae can be written as , where S is the area under consideration satisfying and is the volume velocity. Here the HR with an acoustic impedance Z a 2 is introduced into the interface of the plate and the volume velocity can be split into two parts, , where the first part is the integral of the normal velocity outside the neck of the HR (volume velocity outside the HR) and the second part is the integral of the normal velocity at the entry of the neck of the HR (volume velocity inside the HR). Moreover, because at the subwavelength scale the acoustic pressure and the normal particle vibration velocity outside the neck of the HR are continuous, then and , so . Substituting this into the formula for specific acoustic impedance, the effective specific acoustic impedance of the boundary can be obtained: . If the dissipation loss is neglected, the acoustic impedance of the HR can be expressed as , where ω is the angular frequency and C a and M a are the acoustic capacitance and the acoustic mass of the HR, respectively (see Supplementary Note 2 ). Owing to a large difference in specific acoustic impedance between air and steel, Z s →∞, then . In our two-dimensional (2D) sample, the area of unit cell ( S ) is the period of the HR ( d ). Therefore, the effective acoustic impedance is . 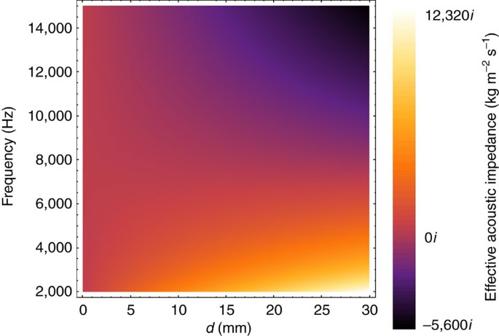Figure 3: Effective acoustic impedance. The effective acoustic impedance is plotted versus the period of the HR (d) and frequency. At low frequency, the effective acoustic impedance is capacitive reactance. At high frequency, the effective acoustic impedance is inductive reactance. Figure 3 presents the effective acoustic impedance versus the period of the HR and frequency. When the resonance condition is met—that is, , then Z a2 =0. This explains how the HR can convert the rigid boundary into a free boundary. Moreover, the impedance analysis procedures are not affected by the length of the centre slit, and so the radiation pattern is irrelevant to the transmission peak of the structure. Figure 3: Effective acoustic impedance. The effective acoustic impedance is plotted versus the period of the HR ( d ) and frequency. At low frequency, the effective acoustic impedance is capacitive reactance. At high frequency, the effective acoustic impedance is inductive reactance. Full size image The acoustic wave equation and the boundary condition can be expressed as and , where the point source (radiation mouth of the central slit) is located at ( x 0 , y 0 ). Through complex calculations, we obtain the Green function of the wave equation in a 2D situation (see Supplementary Note 3 ): Here the time-harmonic factor e − iω t is omitted; k x and are the wave numbers in the x and y directions, respectively, and c 0 and ρ are the speed of sound and density of air, respectively. The Green function includes two items: the first item is the acoustic field caused by the point source and the second item is caused by the virtual source located at ( x 0 , −y 0 ) induced by the boundary. When (that is, ), the acoustic field is the radiation field caused by two point sources with the same phase. When (that is, ), the acoustic field is the radiation field caused by two point sources with opposite phases [26] , which is the dipole pattern. When is relatively low, the acoustic field is the dipole-like shape. When is some other value, the situation becomes more complicated. If the point source is close to the origin point ( x 0 =0, y 0 <<1), equation (1) can be reduced to For a point source in infinite space and located at the original point, it is easy to obtain its plane wave expansion form: Compared with equation (3), equation (2) is multiplied by one more factor, . This factor tailors the scale of each different k x . This is very different from the modulation of k y with different k x (refs 27 , 28 ), which is through designing special material properties in the whole wave region—that is, anisotropic density. We only change the boundary instead of the material properties throughout the whole propagation region, such that keeps unchanged. 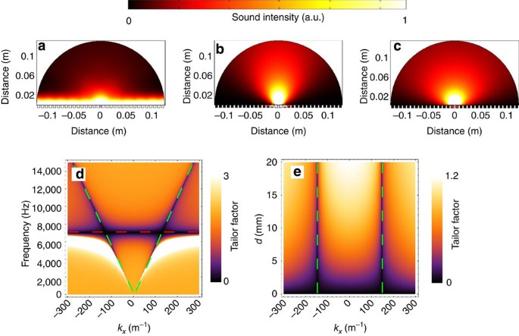Figure 4: Theoretical explanation of effective impedance boundary-induced directivity control. (a–c) Simulated intensity patterns of a plane wave passing decorated sample at 5,800 Hz, 8,600 Hz and 15,000 Hz, respectively. (d) Tailor factor changing with frequency andkx. The red dashed line represents the resonance frequency of the HR and the green dashed line represents the situation in whichkyequals zero. (e) Tailor factor changing with the period of HR andkxatf=8,000 Hz. The green dashed line represents the situation in whichkyequals zero. Figure 4a–c shows the numerical results of the intensity distribution through the decorated sample for 5,800 Hz, 8,600 Hz and 15,000 Hz, respectively. (The resonance frequency of the HR is 7,040 Hz.) Through the analysis above, it can be seen that the acoustic pattern is a dipole-like shape at f =8,600 Hz ( Fig. 4b ). This is because when the frequency is near the resonance frequency of the HR, the effective specific acoustic impedance tends to be zero. We also find that when the frequency is below the resonance frequency ( Fig. 4a ), the intensity is very strong near the interface, which is attributed to the stimulation of the surface wave. In order to explain this phenomenon, we calculated the tailor factor as a function of frequency and k x , as shown in Fig. 4d . The red dash line represents the resonance frequency of the HR and the green dash line represents the situation in which k y equals zero. Below the red dash line and outside but near the region decided by the green dash line, the tailor factor becomes very large. Here is an imaginary number and this is why a strong surface wave is caused. If , the tailor factor tends to be infinitely large. Only when is the condition met. Thus, the surface wave will only be caused when the frequency of the incidence wave is below the resonance frequency of the HR. Above the resonance frequency, no surface wave will be stimulated but the intensity distribution shows a single lobe in the radiation pattern. As the frequency increases, the change rate of the tailor factor is no longer obvious and the directivity worsens due to the fact that the specific acoustic impedance increases with the increase of the frequency. However, the tailor factor becomes zero for all frequencies when k y =0, which is why the radiation pattern can be obtained over a broad bandwidth, as seen in Fig. 4b for f =8,600 Hz and in Fig. 4c for f =15,000 Hz. Figure 4e shows the tailor factor as a function of the period of the HR and k x at f =8,000 Hz. With the increase in period, the change rate of the tailor factor is no longer obvious because the effective specific acoustic impedance is the harmonic mean of the specific acoustic impedance of the boundary and the impedance of the HR. When the period constant increases, the effective impedance increases. Figure 4: Theoretical explanation of effective impedance boundary-induced directivity control. ( a – c ) Simulated intensity patterns of a plane wave passing decorated sample at 5,800 Hz, 8,600 Hz and 15,000 Hz, respectively. ( d ) Tailor factor changing with frequency and k x . The red dashed line represents the resonance frequency of the HR and the green dashed line represents the situation in which k y equals zero. ( e ) Tailor factor changing with the period of HR and k x at f =8,000 Hz. The green dashed line represents the situation in which k y equals zero. Full size image Influence of the number of HRs on radiation pattern Actually, the number of HRs decorated on the sample will influence the total radiation pattern effect [29] . 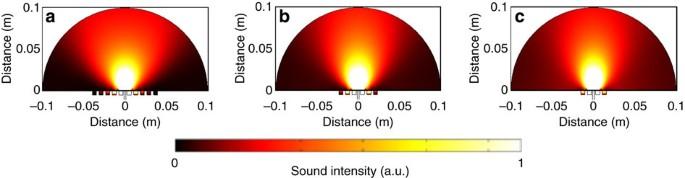Figure 5: Influence of the number of HRs on directivity. (a) Intensity pattern for plane wave through the sample with five HRs in each sides. (b) Intensity pattern for plane wave through the sample with three HRs in each sides. (c) Intensity pattern for plane wave through the sample with two HRs in each sides. Figure 5a–c shows the intensity field at f =8,500 Hz for five, three and two HRs on each side. It should be noted that the period of the HR is d =8 mm and the wavelength at f =8,500 Hz is λ =4 cm. That is to say, the total length of the decorated surface used to control the wave pattern is 8 cm (2 λ ), 4.8 cm (1.2 λ ) and 3.2 cm (0.8 λ ). Comparing Figs 5a and 1c , we find that the radiation pattern of each is almost the same. However, as the number of HRs continues to decrease, the directivity worsens but radiation pattern is maintained. This is quite different from the results reported previously because the total width of the decorated sample needed to realize radiation pattern in that study should be larger than 11 λ (ref. 30 )—otherwise, the directional pattern disappears. As the total length of the decorated surface needed to obtain radiation pattern is so short, we used an intersection angle of 90° on the sample surface, as shown in Fig. 6a , and the number of HRs used is six on each side. It should be noted that the width of the open mouth of the intersection angle is only 6.8 cm. The experimental facility is shown in Fig. 6b and the detail of the experimental method is provided in the Methods below. The experimental result of full-range intensity field pattern is shown in Fig. 6c in the dB scale. This agrees well with simulations as shown in Fig. 6d . Please note that the experimental region in the y direction is from 0.05 m due to the finite size of the microphone and the sample. As the effective acoustic impedances of the two boundaries tended to be zero when the frequency was near the resonance of the HRs, the intensity distribution was quadrupole-shaped. In order to compare the effect caused by the HRs, we provide the experimental results and simulations of the full-range intensity field patterns for the sound wave travel through the sample without an HR, as shown in Fig. 6e,f . It is clear that changing the effective acoustic impedance boundary will significantly improve the directivity of the wave but without causing any sidelobe. It should be noted that the intersection can be all degrees, and smaller angles produce better directivity. Figure 5: Influence of the number of HRs on directivity. ( a ) Intensity pattern for plane wave through the sample with five HRs in each sides. ( b ) Intensity pattern for plane wave through the sample with three HRs in each sides. ( c ) Intensity pattern for plane wave through the sample with two HRs in each sides. 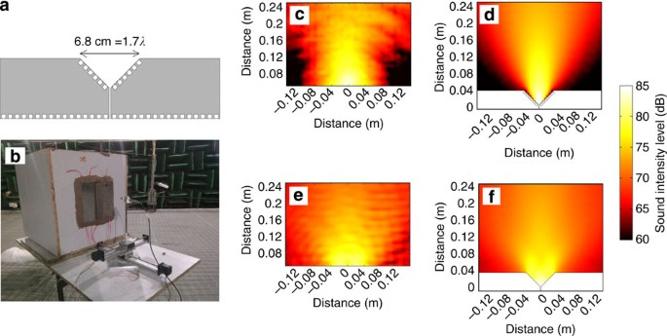Figure 6: Experimental observation of the intensity pattern for the sound wave travelling through the flanked structure. (a) Top views of the sample with 90° intersection angle and six HR on each flanks. (b) Experimental facility. (c) Experimental and (d) simulated results of intensity patterns of a plane wave passing the sample inFig. 6a. (e) Experimental and (f) simulated results of intensity patterns of a plane wave passing the sample without HR on each flanks. Full size image Figure 6: Experimental observation of the intensity pattern for the sound wave travelling through the flanked structure. ( a ) Top views of the sample with 90° intersection angle and six HR on each flanks. ( b ) Experimental facility. ( c ) Experimental and ( d ) simulated results of intensity patterns of a plane wave passing the sample in Fig. 6a . ( e ) Experimental and ( f ) simulated results of intensity patterns of a plane wave passing the sample without HR on each flanks. Full size image The realization of collimated beam has been reported by using phononic crystal [31] —that is, the collimated beam is realized when the wavelength is the same order as the lattice constant. Here we provide a feasible way to realize acoustic collimation beam in subwavelength scale—that is, the collimated beam can be realized when the lattice constant is much smaller than the wavelength, which can be utilized to realize device miniaturization. Equation (2) provides a flexible way to control radiation pattern. If piezo-diaphragm is introduced to the bottom of the cavity of each HR, passive HR is converted to be active HR. One of the characteristics of active material is that its resistance can be negative [32] . If suitable piezo-diaphragm is chosen and voltage is well applied to the piezo-diaphragm, desired effective impedance can be obtained [33] , [34] . In our simulation, we set the effective specific impedance of the boundary caused by active HR to be =−426 kg m −2 s −1 , and the density and sound speed of air are ρ =1.25 kg m −3 and c 0 =343 m s −1 , respectively. Owing to the fact that effective specific impedance is negative, the value of tends to be very small when ( k x =0). Therefore, the tailor factor tends to be very large when k x =0 but very small when k y =0. 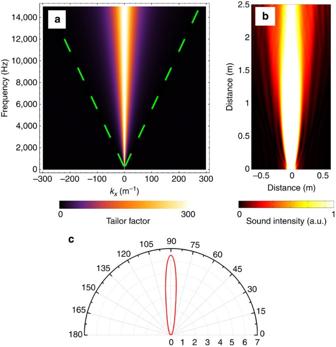Figure 7: Beam collimation. (a) Tailor factor change with frequency andkxwhen=−426 kg m−2s−1. The green dashed line represents the situation in whichkyequals zero. (b) Numerical intensity patterns of the wave with negative impedance boundary. (c) Theoretical calculated directivity pattern of the wave with negative impedance boundary. Figure 7a presents the tailor factor as a function of frequency and k x . It is very large when k x =0 and is restrained when k y =0. Therefore, collimation beam can be obtained in such effective boundary. Figure 7b,c presents the numerical intensity distribution of the wave and theoretical calculated directivity pattern in the far field, respectively. Far from 2.5 m (60 wavelength), the wave is still with good directivity. Moreover, the collimated beam is without any sidelobe. Figure 7: Beam collimation. ( a ) Tailor factor change with frequency and k x when =−426 kg m −2 s −1 . The green dashed line represents the situation in which k y equals zero. ( b ) Numerical intensity patterns of the wave with negative impedance boundary. ( c ) Theoretical calculated directivity pattern of the wave with negative impedance boundary. Full size image In conclusion, with constructing a new type of structure, we observed the dipole-like radiation induced by tailoring the wave vector. It is worth noting that the exotic dipole-like radiation phenomenon is accompanied by high radiation efficiency and relatively wide bandwidth. Moreover, the dipole-like radiation is without any sidelobe or fingerprint of a running surface wave scattered by the structure. Prospective applications of this mechanism for achieving directional radiation in products such as high-gain loud speakers and ultrasonic medical instrumentation can be expected. Acoustic measurements Our experiment was carried in the anechoic chamber in order to eliminate the influence of the reflected waves. The propagation medium of the acoustic wave was air. In the experiment, a sound insulation box is used to avoid the diffraction from the edge of the sample. When measuring the intensity field pattern of the sound wave travel through the sample, a loudspeaker is put in the sound insulation box. The pressure signal was picked up by a free-field 1/2-inch microphone. The microphone is fixed in the stepper motor controlled by the computer, as shown in Fig. 6b . How to cite this article: Quan, L. et al. Effective impedance boundary optimization and its contribution to dipole radiation and radiation pattern control. Nat. Commun. 5:3188 doi: 10.1038/ncomms4188 (2014).